Kinetic resolution of cyclic benzylic azides enabled by site- and enantioselective C(sp3)–H oxidation Catalytic nonenzymatic kinetic resolution (KR) of racemates remains one of the most powerful tools to prepare enantiopure compounds, which dominantly relies on the manipulation of reactive functional groups. Moreover, catalytic KR of organic azides represents a formidable challenge due to the small size and instability of the azido group. Here, an effective KR of cyclic benzylic azides through site- and enantioselective C(sp 3 )–H oxidation is described. The manganese catalyzed oxidative KR reaction exhibits good functional group tolerance, and is applicable to a range of tetrahydroquinoline- and indoline-based organic azides with excellent site- and enantio-discrimination. Computational studies elucidate that the effective chiral recognition is derived from hydrogen bonding interaction between substrate and catalyst. Catalytic nonenzymatic kinetic resolution (KR) of racemates is one of the most powerful and practical tools to prepare valuable enantiopure targets, especially in cases where other methods are not possible or provide insufficient enantiocontrol [1] , [2] , [3] , [4] , [5] . Chiral organic azides are versatile synthetic precursors for a range of nitrogen-containing molecules and have found dramatically expanded utility in medicine, biology, and material science [6] , [7] , [8] , [9] , [10] , [11] , [12] , [13] , [14] , [15] . However, catalytic KR to provide optically pure azides has remained elusive, principally due to two essential features of the azido moiety: (1) the instability hampering the design of new reactivity with excellent chemoselectivity; (2) the small size hampering the achievement of effective chiral recognition [16] , [17] , [18] , [19] , [20] , [21] . Existing isolated examples always focused on manipulating the azido moiety through azide–alkyne cycloaddition (AAC) [22] , [23] , [24] , [25] , [26] (Fig. 1A ) or extra reactive functional groups preinstalled in substrates (Fig. 1B ) [27] , [28] , which typically suffer from the use of excess azide substrates, poor chiral recognition, and narrow substrate scope. Developing an effective KR of organic azides relying on the reactivity of C(sp 3 )–H bonds would be highly desired [29] . Fig. 1: Overview of KR methods to prepare chiral organic azides. A KR of benzylic azides through azide–alkyne cycloaddition. B KR of allylic azides through asymmetric dihydroxylation of alkene. C KR of cyclic benzylic azides through asymmetric C(sp 3 )−H oxidation. Full size image Nonenzymatic site- and enantioselective oxidation of ubiquitous C(sp 3 )−H bonds with a general scope and predictable selectivity represents a paradigm shift in the standard logic of organic synthesis [30] , [31] . However, such research topic has remained a formidable challenge, and current studies typically suffer from moderate enantioselectivity, low substrate conversion, and narrow substrate scope [32] , [33] , [34] , [35] , [36] , [37] , [38] , [39] , [40] , [41] , [42] , [43] , [44] . In particular, catalytic KR through C(sp 3 )–H oxidation dominantly focused on secondary alcohols [45] , [46] , [47] , [48] , [49] , [50] , [51] , [52] and amines [53] , [54] due to their high and well-known oxidized reactivity together with the presence of a strong interaction site with catalyst for efficient chiral recognition [55] , [56] . To our knowledge, selective oxidation of C(sp 3 )−H bond adjacent to azido moiety remains elusive. Moreover, organic azide lacks such an effective interaction site to direct substrate to an ideal location in the transition state. Therefore, chiral recognition of chemically similar C(sp 3 )−H bonds adjacent to azido group of two enantiomers would be difficult to accomplish. Herein, we report the KR of organic azides through site- and enantioselective C(sp 3 )–H bond oxidation (Fig. 1C ). First, given the significance of benzo-fused nitrogen-containing heterocycles in modern pharmacology, we choose a range of racemic benzylic azides bearing such skeletons as substrates. Second, we select the readily modifiable salen as the basal ligand to search for suitable base-metal catalyst. Third, varying the protecting group on the nitrogen moiety might also provide an opportunity to tune the chiral recognition. Based on these considerations, a range (36 examples) of cyclic benzylic azides participate in oxidative KR with good to excellent selectivity factors ( s up to 95). 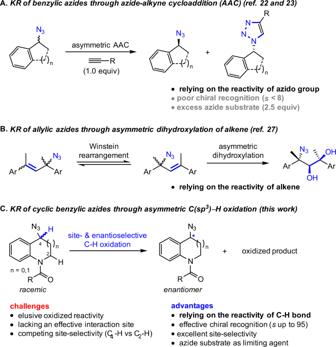Fig. 1: Overview of KR methods to prepare chiral organic azides. AKR of benzylic azides through azide–alkyne cycloaddition.BKR of allylic azides through asymmetric dihydroxylation of alkene.CKR of cyclic benzylic azides through asymmetric C(sp3)−H oxidation. Reaction condition optimization The oxidative KR of tetrahydroquinoline (THQ) based organic azide rac- 1a was selected as the model reaction for optimization (Table 1 ). In the presence of PhIO as the oxidant, no reaction was observed for either chiral Fe(salen) C1 or Co(salen) C2 (entry 1). Chiral Mn(salen) C3 exhibited good oxidation catalysis reactivity, though poor chiral recognition was obtained (entry 2). Oxidation proceeded with excellent site selectivity at the C 4 –H bond adjacent to azido moiety over C 2 –H bond α to amide motif, affording azine 2a as oxidized product. Mn(salen) C4 having cyclohexanediamine skeleton provided better results than C3 with 1,2-diphenyl-1,2-ethanediamine (entry 3). Careful examination of the substituent effects on the basal salen ligand revealed C12 with 2,4-difluorophenyl moieties at C3(3’) sites to be optimal (entries 4–10). Other oxidants such as H 2 O 2 and NaClO afforded inferior oxidation reactivity (entry 11). Addition of PhIO as eight equal portions in 30 min intervals was beneficial for achieving an extremely high level of chiral discrimination, and ( S )- 1a was isolated in 48% yield with 98% ee ( s = 91, entries 12 and 13). Table 1 Reaction condition optimization a . Full size table Substrate scope The scope of oxidative KR of THQ-based organic azides was explored (Fig. 2 ). In general, both electron-rich and -deficient THQ skeletons were well tolerated, as demonstrated by effective access to optically pure 1a - 1m with good to excellent selectivity factors ( s = 32–91). Resolution efficiency was not impaired for reaction on a 0.5 mmol scale. Common functional groups, including halide, acetate, silyl ether, benzoate, and triflate, were tolerated for further manipulation. Racemic THQ-based organic azides bearing two stereocenters were also suitable components with good enantio-discrimination. Oxidative KR of cis -2,4-disubstituted rac- 1n proceeded, furnishing (2 R ,4 S )- 1n in 47% yield with 92% ee (The absolute configuration of recovered 1n was determined by X-ray diffraction analysis. See the Supporting Information for details). The reaction was not sensitive to the steric hindrance of C 2 -substituents, as demonstrated by access to respective enantiopure 1o - 1u with good selectivity factors ( s = 20–35). Fig. 2: Kinetic resolution of THQ-based organic azides. Conditions: rac- 1 (0.1 mmol), PhIO (0.08 mmol, addition as 8 portions in 30-min intervals over 3.5 h), and C12 (5 mol%) in ethyl acetate (1.0 ml) at rt for 4 h. a Reaction with 0.5 mmol rac- 1 . b Reaction with 1.0 gram of rac- 1 . Full size image Indoline represents the other type of biologically important benzo-fused nitrogen-containing heterocycle. Accordingly, the applicability of the oxidative KR strategy in enantioselective access to indoline-based azides was next explored (Fig. 3 ). When Mn(salen) C7 was used as catalyst, oxidative KR of cyclic benzylic azide rac- 3a proceeded, furnishing 2-aminobenzonitrile 4a as oxidized product together with recovered ( S )- 3a in 48% yield with 96% ee ( s = 65) (The absolute configuration of recovered 3a was determined by X-ray diffraction analysis. See the Supporting Information for details). Notably, the reaction exhibited excellent site selectivity at the C 3 –H bond adjacent to azido moiety over C 2 –H bond α to amide motif. Indolines rac- 3b - 3h bearing electronically varied groups around the arene moiety were tolerated with a high level of chiral recognition ( s = 36–95). Selectivities were not impaired for reaction on a 0.5 mmol scale. Substrates bearing other N -acyl groups, such as propanoyl ( 3i ) and butyryl ( 3j ), were also tolerated, though no reaction was observed for pivaloyl one ( 3k ). Fig. 3: Kinetic resolution of indoline-based organic azides. Conditions: rac- 3 (0.1 mmol), PhIO (0.08 mmol, addition as 8 portions in 30-min intervals over 3.5 h), and C7 (5 mol%) in ethyl acetate (1.0 ml) at rt for 4 h. a Reaction with 0.5 mmol rac- 3 . Full size image Synthetic applications Manipulating the azido moiety through copper-catalyzed AAC would allow facile integration of the other biologically important molecules into N -heterocycles for drug discovery. For example, vitamin E derivative ( 5 ) with potent antioxidation activity and estrone derivative ( 7 ) for treating abnormalities associated with menopause are efficiently installed into THQ skeleton using triazole as a linker, respectively (Fig. 4 ). Fig. 4: Synthetic applications. A CuSO 4 -catalyzed AAC of optically pure THQ-based organic azide and vitamin E derivative. B CuI-catalyzed AAC of optically pure THQ-based organic azide and estrone derivative. Full size image Mechanistic and DFT studies Control experiments were conducted to get a preliminary understanding of the reaction mechanism (Fig. 5 ). The relationship between ee values of Mn(salen) catalyst and recovered substrate was explored, showing that the enantioselectivity of recovered 3a is proportional to the ee of C7 (Fig. 5A ). The absence of nonlinear effects indicated that the reaction might not involve heterochiral aglomerates [57] , [58] . No reaction was observed for stoichiometric Mn(salen) C12 mediated reaction in the absence of PhIO, suggesting that oxoMn(V) might be the species in charge of C–H oxidation (Fig. 5B ). A competition deuterium kinetic isotope effect (KIE) study, using a mixture of rac- 1a and [D]-rac- 1a , revealed a KIE of 2.7 (Fig. 5C ). The observation implied that C−H bond cleavage might be involved in the rate-determining step. The substituent effect of different acyl groups on THQ-based azides was explored (Fig. 5D ). Several aspects of the data merit further comment. Firstly, no reaction was observed for N -acyl substituted 9a . Secondly, the oxidized reactivity was gradually enhanced as the increasing numbers of methyl groups at α-position of the carbonyl moiety ( 9a - 9c and 1a ). Thirdly, the oxidative reactivity was lost when placing an oxygen atom between the carbonyl and t Bu groups. In general, more sterically hindered substrates should exhibit lower reactivity than that of less sterically hindered ones. We speculated that the opposite trend observed for THQ-based substrates in Fig. 5D might originate from the non-covalent interaction between the α-alkyl group of carbonyl moiety and Mn(salen) catalyst. The deuteration effect of the N -acyl moiety of indoline-based substrates was next evaluated (Fig. 5E ). No oxidative conversion was observed for [D]- 3a , indicating that the sp 3 C–H bond at α-position of carbonyl motif is crucial to the reactivity of substrate 3a . Fig. 5: Control experiments. A Plot of enantiomeric excess of recovered 3a versus the enantiomeric excess of C7 at 20% conversion. The dotted line symbolized the linear correlation. B Stoichiometric Mn(salen) C12 mediated control experiment in the absence of PhIO. C The intermolecular kinetic isotope effect. D The N -acyl substituent effect for THQ-based azides. E Deuterated control experiment of indoline-based azide. Full size image According to the generally accepted mechanism of manganese-catalyzed C(sp 3 )−H oxidation and the control experiments, a plausible mechanistic pathway for oxidative KR of benzylic azides was suggested (Fig. 6 ) [59] . Chiral Mn III catalyst is first oxidized by PhIO affording oxoMn V intermediate. THQ rac- 1a underwent hydrogen atom transfer (HAT) to oxoMn V , giving benzylic radical 10 and Mn IV −OH. Finally, azide 10 decomposed by losing molecular nitrogen to form iminyl radical 11 , which immediately dimerized to provide 2a [60] . Mn IV −OH dimerized by releasing H 2 O to generate μ -oxo bridged dimer Mn IV OMn IV , which might undergo disproportionation reaction regenerating Mn III precursor and oxoMn V species for the catalytic cycle [61] , [62] , [63] . Based on the absolute configuration of recovered THQs, ( R )- 1a should be oxidized more preferentially than ( S )- 1a . With respect to the oxidative KR of indoline-based benzylic azides, rac- 3a might proceed through a similar HAT process to oxoMn V species producing benzylic radical 12 , which underwent azide collapse followed by C−C bond cleavage forming radical 14 . Alkyl radical 14 underwent oxygen rebound with Mn IV −OH followed by hemiaminal decomposition, generating 2-aminobenzonitrile 4a together with Mn III precursor for the catalytic cycle. Based on the absolute configuration of recovered indolines, ( R )- 3a should be oxidized more preferentially than ( S )- 3a . Fig. 6: Proposed reaction mechanism. The possible reaction pathway based on our studies and the previous literatures. Full size image To elucidate the origin of the high level of chiral recognition of azide rac- 1a , density functional theory (DFT) calculations were performed for the stereo-determining HAT process (Fig. 7 ). The Gibbs free energies of corresponding transition states follow the spin ordering of triplet < quintet < singlet, and the triplet state was determined to be the ground state (see Table S1 in the Supporting Information ). 3 TS R is 1.8 kcal/mol more favorable than 3 TS S , which is consistent with experimentally observed stereoselectivity. The effective chiral recognition arises from additional CH···F hydrogen bonding interaction between tert -butyl group of ( R )- 1a and 2,4-difluorophenyl moiety of catalyst C12 in 3 TS R . This CH···F hydrogen bonding interaction is further confirmed by independent gradient model analysis [64] . Fig. 7: Geometries and the relative Gibbs free energies of stereoselectivity-determining transition states. Trivial hydrogen atoms are omitted for clarity. The isosurface of IGM analysis is 0.005. The bond distances are given in Å. All energies are given in kcal/mol. Full size image In this work, the KR of organic azides through site- and enantioselective C(sp 3 )–H oxidation is described. 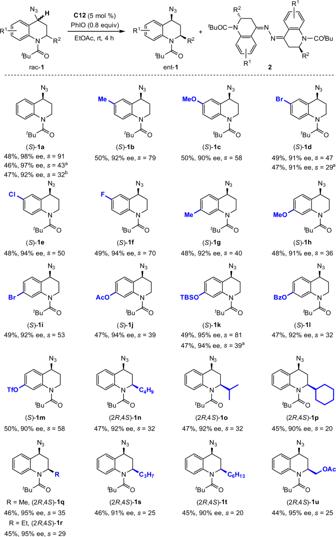Fig. 2: Kinetic resolution of THQ-based organic azides. Conditions: rac-1(0.1 mmol), PhIO (0.08 mmol, addition as 8 portions in 30-min intervals over 3.5 h), andC12(5 mol%) in ethyl acetate (1.0 ml) at rt for 4 h.aReaction with 0.5 mmol rac-1.bReaction with 1.0 gram of rac-1. The practical manganese catalyzed reaction exhibits good functional group tolerance, and is applicable to a variety of cyclic benzylic azides bearing pharmacologically significant nitrogen-containing heterocycle skeletons with extremely efficient site- and enantio-discrimination. The usefulness of products has also been demonstrated in synthetic applications. Detailed computational studies elucidate the origins of effective chiral recognition involving a hydrogen bonding interaction between substrate and catalyst. This strategically different approach would unlock opportunities for topologically straightforward synthetic planning for KR reactions relying on the reactivity of C(sp 3 )–H bonds. 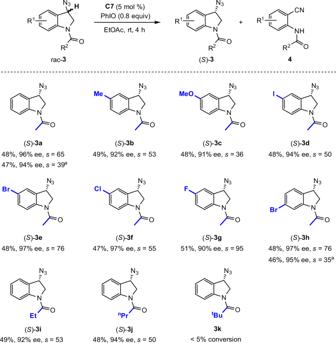Fig. 3: Kinetic resolution of indoline-based organic azides. Conditions: rac-3(0.1 mmol), PhIO (0.08 mmol, addition as 8 portions in 30-min intervals over 3.5 h), andC7(5 mol%) in ethyl acetate (1.0 ml) at rt for 4 h.aReaction with 0.5 mmol rac-3. General procedure To a solution of rac- 1a (0.1 mmol, 1.0 equiv) in ethyl acetate (1.0 ml) was added C12 (0.005 mmol, 0.05 equiv) at room temperature. 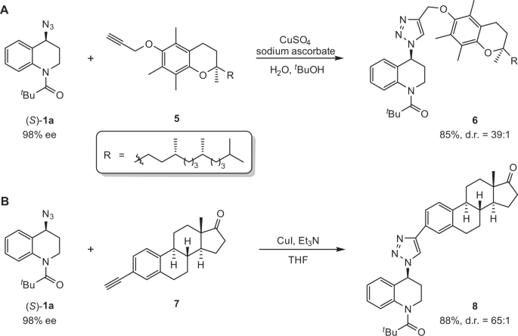Fig. 4: Synthetic applications. ACuSO4-catalyzed AAC of optically pure THQ-based organic azide and vitamin E derivative.BCuI-catalyzed AAC of optically pure THQ-based organic azide and estrone derivative. 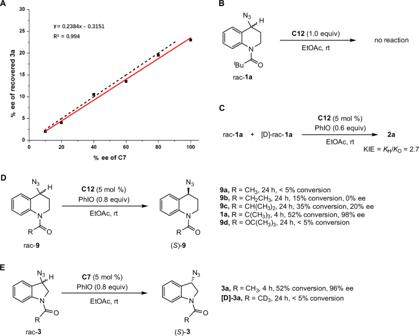Fig. 5: Control experiments. APlot of enantiomeric excess of recovered3aversus the enantiomeric excess ofC7at 20% conversion. The dotted line symbolized the linear correlation.BStoichiometric Mn(salen)C12mediated control experiment in the absence of PhIO.CThe intermolecular kinetic isotope effect.DTheN-acyl substituent effect for THQ-based azides.EDeuterated control experiment of indoline-based azide. 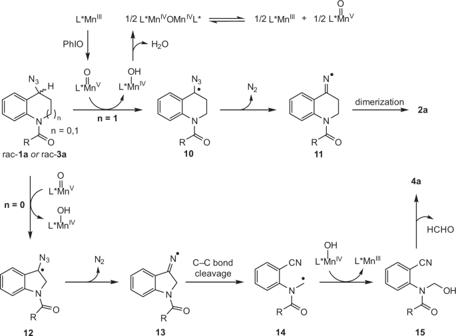Fig. 6: Proposed reaction mechanism. The possible reaction pathway based on our studies and the previous literatures. 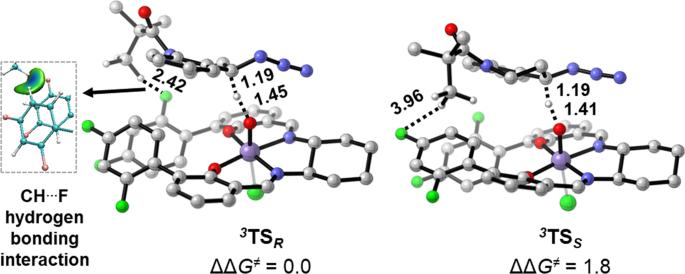Fig. 7: Geometries and the relative Gibbs free energies of stereoselectivity-determining transition states. Trivial hydrogen atoms are omitted for clarity. The isosurface of IGM analysis is 0.005. The bond distances are given in Å. All energies are given in kcal/mol. Then PhIO (0.08 mmol, 0.8 equiv) was added as eight portions in 30-min intervals over 3.5 h. After that, the solvent was removed under vacuum and the residue was purified by flash chromatography on silica gel using ethyl acetate/petroleum ether as eluent to give the product ( S )- 1a .